Dietary restriction protects against experimental cerebral malaria via leptin modulation and T-cell mTORC1 suppression Host nutrition can affect the outcome of parasitic diseases through metabolic effects on host immunity and/or the parasite. Here we show that modulation of mouse immunometabolism through brief restriction of food intake (dietary restriction, DR) prevents neuropathology in experimental cerebral malaria (ECM). While no effects are detected on parasite growth, DR reduces parasite accumulation in peripheral tissues including the brain, and increases clearance in the spleen. Leptin, a host-derived adipokine linking appetite, energy balance and immune function, is required for ECM pathology and its levels are reduced upon DR. Recombinant leptin abrogates DR benefits, while pharmacological or genetic inhibition of leptin signalling protects against ECM. DR reduces mTORC1 activity in T cells, and this effect is abrogated upon leptin administration. Furthermore, mTORC1 inhibition with rapamycin prevents ECM pathology. Our results suggest that leptin and mTORC1 provide a novel mechanistic link between nutrition, immunometabolism and ECM pathology, with potential therapeutic implications for cerebral malaria. Host nutritional status can have a major influence on immune function in part because nutrient and pro-inflammatory signals are integrated through common evolutionarily conserved signal transduction molecules [1] , [2] . Mechanistic target of rapamycin complex 1 (mTORC1), for example, can respond to the presence of nutrients and growth factors, but also pro-inflammatory hormones including the adipokine leptin [3] , [4] , [5] , [6] , [7] . Leptin is secreted by white adipocytes in proportion to the percent body fat [8] . Leptin acts both centrally and peripherally to reduce appetite and increase energy expenditure, in part through modulation of mTORC1 activity. Leptin can also act on innate and adaptive immune cells, including T lymphocytes, to increase expression of cell surface adhesion molecules and chemokine receptors including P-selectin ligands and CXCR3 downstream of mTORC1 activation [9] , [10] . Dietary restriction (DR), defined as reduced food intake without malnutrition, is best recognized for its ability to extend lifespan in most organisms tested [11] . DR also confers benefits on metabolic health (glucose homeostasis, lipid handling) and increased resistance to a variety of different stressors (heat shock, oxidative stress and so on) [12] . On the molecular level, DR is not well understood but is thought to function at least in part through inhibition of mTORC1 based on data from lower organisms [13] . DR also reduces adiposity and corresponding leptin levels, thus potentially further reducing mTORC1 activation status [3] . Partial mTORC1 inhibition with the allosteric inhibitor rapamycin recapitulates some benefits of DR, including extended longevity [14] , [15] . Although DR has broad anti-inflammatory effects in a number of contexts (for example, lipopolysaccharide challenge, models of sterile inflammation) [12] , the impact of DR on immunometabolism in the context of infectious diseases involving both innate and adaptive immune components remains poorly characterized. Cerebral malaria (CM) is the most dangerous sequela of Plasmodium falciparum infection resulting in high mortality and morbidity [16] . While little is known about the pathophysiology of CM in humans, models of experimental CM (ECM) caused by infection of susceptible mice, including C57BL/6 mice, with the P. berghei ANKA parasite, have provided important clues. ECM is a severe neurovascular disease characterized by disruption of the blood–brain barrier (BBB) followed by seizures, coma and death [17] . Vascular breakdown is mediated by antigen-specific cytotoxic CD8+ T lymphocytes activated in the spleen and recruited to the brain in the presence of parasitized red blood cells (RBCs) [18] , [19] . While malarial infection can clearly be affected by nutritional status of the host, whether the extremes of obesity and starvation are protective or detrimental to disease outcome remains poorly understood [20] , [21] . Here we report that brief periods of DR starting on the day of infection prevent severe ECM symptoms and death in mice through modulation of leptin levels and mTORC1 activation in CD4+ and CD8+ T cells, resulting in increased numbers of active T cells in the spleen and less in the brain late in infection when severe neurological symptoms arise. Pharmacological inhibition of either leptin signalling with a mutant peptide, or downstream mTORC1 signalling with rapamycin, blocks ECM symptoms and reduces mortality, thus revealing two novel host targets for potential treatment of CM. DR modulates susceptibility to ECM Mice were subject to varying degrees of DR (10–50%) relative to ad libitum (AL)-fed controls starting 7 days before infection on day 0 with P. berghei ANKA-infected RBCs ( Fig. 1a–e ), or restricted at 40% starting at different time points (−7, −4, −2, 0 or +2 days of infection, Fig. 1f–j ). Restricted mice were fed a fixed amount of food daily until the end of the experiment on day 10–12 after infection ( Fig. 1a,f ) resulting in the loss of body weight proportional to food restriction ( Fig. 1b,g ). Sickness-related anorectic behaviour (voluntary-reduced food intake) was delayed and mitigated in DR groups relative to AL controls ( Fig. 1a,f ). The percentage of infected RBCs in peripheral blood did not correlate with food restriction ( Fig. 1c,h ). Most infected mice in the AL group died of neurological symptoms or were killed according to humane end points between days 6 and 12 after infection. Survival was significantly improved by DR, often reaching 100% protection without symptoms of ECM by day 12 after infection ( Fig. 1d,i ). However, when 40% DR was started 2 days after infection, food intake was similar to AL mice and no protection was obtained ( Fig. 1f,i ). The cumulative survival percentage 12 days after infection from multiple independent experiments confirmed optimal survival with 40% food restriction starting the day of infection ( Fig. 1e,j ). Furthermore, these results demonstrate the requirement of DR within 2 days of infection in order to afford protection. All subsequent experiments were thus performed comparing AL to 40% DR starting the day of infection. 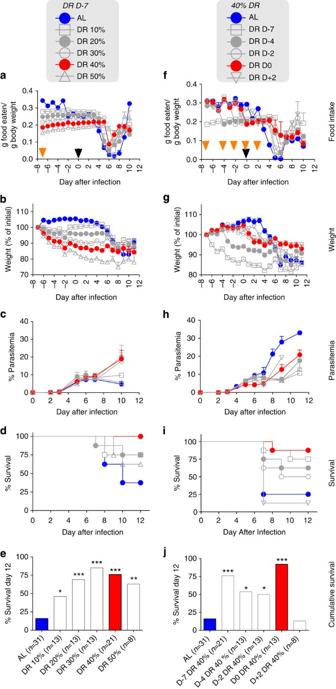Figure 1: Dietary restriction modulates susceptibility to ECM. Representative experiments to examine the dose–response to DR (a–e) and the kinetics of onset of DR benefits (f–j). Eight mice per group in two cages were food-restricted by 10–50% as indicated (DR 10–50%) relative to AL-fed controls for 7 days (a–d, DR D-7) or 40% restricted from the indicated day (f–i, 40% DR). All mice were infected on day 0 (black arrowhead) and monitored until day 10–12 after infection; orange arrowheads indicate onset of food restriction. (a,f)Food intake.Average daily food consumption of the indicated group expressed as grams of food eaten per total weight of animals in that cage. (b,g)Weight.Body weight was measured daily starting 7 days before the infection and expressed as a percentage of starting weight. (c,h)Peripheral parasitemia.The percentage of infected RBCs in circulation was assessed by flow cytometry on the indicated day after infection. (d,i)Survival.Kaplan–Meier curves indicative of survival of infected mice exposed to different levels of DR. (e,j)Cumulative survival.Percentage of survival 12 days after infection. Data from two to four independent experiments per group were pooled, withnindicating total number of mice in each group. Asterisks represent significance of the corresponding Kaplan–Meier survival curves by log-rank test relative to the AL group; *P<0.05, **P<0.01, ***P<0.001. Values are the means and error bars represent s.e.m. Figure 1: Dietary restriction modulates susceptibility to ECM. Representative experiments to examine the dose–response to DR ( a – e ) and the kinetics of onset of DR benefits ( f – j ). Eight mice per group in two cages were food-restricted by 10–50% as indicated (DR 10–50%) relative to AL-fed controls for 7 days ( a – d , DR D-7) or 40% restricted from the indicated day ( f – i , 40% DR). All mice were infected on day 0 (black arrowhead) and monitored until day 10–12 after infection; orange arrowheads indicate onset of food restriction. ( a , f ) Food intake. Average daily food consumption of the indicated group expressed as grams of food eaten per total weight of animals in that cage. ( b , g ) Weight. Body weight was measured daily starting 7 days before the infection and expressed as a percentage of starting weight. ( c , h ) Peripheral parasitemia. The percentage of infected RBCs in circulation was assessed by flow cytometry on the indicated day after infection. ( d , i ) Survival. Kaplan–Meier curves indicative of survival of infected mice exposed to different levels of DR. ( e , j ) Cumulative survival. Percentage of survival 12 days after infection. Data from two to four independent experiments per group were pooled, with n indicating total number of mice in each group. Asterisks represent significance of the corresponding Kaplan–Meier survival curves by log-rank test relative to the AL group; * P <0.05, ** P <0.01, *** P <0.001. Values are the means and error bars represent s.e.m. Full size image In principle, even mild DR could reduce nutrient availability to the parasite, thus affecting outcome based on reduced parasite growth or development. However, we found no correlation between protection and peripheral parasite growth ( Supplementary Fig. 1a–d ), nor any differences in parasite development within infected RBCs ( Supplementary Fig. 1e ). Furthermore, no evidence was found of glucose or free amino-acid limitations in the serum of infected DR animals relative to AL controls ( Supplementary Fig. 1f–k ), or differences in host haematocrit or platelets as a function of diet ( Supplementary Fig. 1l,m ). These data strongly suggest nutrient/energy availability in food-restricted hosts was unlikely to be limiting for parasite growth or development. Reduction of brain pathology by DR Accumulation of parasitized RBCs in the brain is necessary for the induction of neurological symptoms in the ECM model [22] , [23] . We hypothesized that food restriction might afford protection against neurological complications by modulating accumulation of infected RBCs in the brain. To test this, we injected luciferase-expressing P. berghei ANKA parasites [24] into AL-fed or -restricted mice and determined the degree of parasite accumulation by quantifying luciferase activity in the extracts of brain following perfusion to remove infected RBCs in circulation. Using this novel and sensitive methodology, we consistently observed a significant increase in luciferase activity only in the brain extracts from the AL group and only by day 6, when severe neurological symptoms arise ( Fig. 2a ). Consistent with the suppression of parasite accumulation by DR, quantitative PCR (qPCR) analysis suggested reduced parasite 18S rRNA in brains of DR versus AL mice ( Fig. 2b ). The onset of severe neurological symptoms on day 6 post infection also correlated with the appearance of histopathological abnormalities in the brain including small parenchymal haemorrhages scattered throughout the brain cortex, but predominantly in thalamic structures ( Supplementary Fig. 2a ) and in the cerebellar granule layer ( Supplementary Fig. 2b ). Subarachnoid clumping of RBCs with histopathological evidence of meningitis ( Supplementary Fig. 2b ) and leukostasis in the hippocampal microvasculature ( Supplementary Fig. 2c ) were also observed. 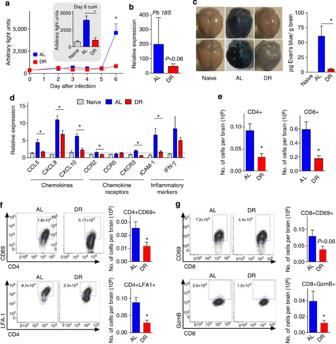Figure 2: Dietary restriction reduces brain parasite accumulation and immunopathology. (a) Luciferase activity from brain extracts of AL or 40% DR mice infected with transgenic luciferase-expressingP. bergheiANKA killed on the indicated day. Luciferase activity indicative of parasite burden is expressed in arbitrary light units. A representative experiment with four animals per group is shown. Inset: cumulative data pooled from independent experiments showing luciferase activity in the brains of naive, AL and DR mice on day 6 after infection. Asterisk indicates the significance of the difference between the indicated groups according to a Mann–Whitney test; *P<0.05. (b) Relative parasite 18S rRNA expression in the brain of AL and DR mice (n=4 per diet group) 6 days after infection as determined by qPCR with aPvalue between AL and DR groups as indicated according to a Mann–Whitney test. (c) Naive, AL or DR mice (n=4 per group) were injected with Evan’s blue and the leakage of the dye into the cerebral tissue representing disruption of BBB was qualitatively (left) and quantitatively (right) assessed on day 6 after infection. A representative experiment is shown. Asterisk indicates the significance of the difference between the indicated groups according to a Mann–Whitney test; *P<0.05. (d) Relative gene expression of chemokines, chemokine receptors and inflammatory markers as indicated in the brain on day 6 after infection of the indicated dietary group as measured by qPCR. Representative experiments with four mice per group are shown. Asterisks indicate the significance of the difference between AL and DR for a given gene according to a Mann–Whitney test; *P<0.05. (e–g) Numbers of total (e) and activated (f,g) CD4+ and CD8+ T lymphocytes with representative dot plots from brains of mice (n=4 per group) of the indicated dietary groups on day 6 after infection following perfusion as determined by FACS. Asterisks indicate the significance of the difference between groups according to a Mann–Whitney test; *P<0.05. Values are means+s.e.m. Figure 2: Dietary restriction reduces brain parasite accumulation and immunopathology. ( a ) Luciferase activity from brain extracts of AL or 40% DR mice infected with transgenic luciferase-expressing P. berghei ANKA killed on the indicated day. Luciferase activity indicative of parasite burden is expressed in arbitrary light units. A representative experiment with four animals per group is shown. Inset: cumulative data pooled from independent experiments showing luciferase activity in the brains of naive, AL and DR mice on day 6 after infection. Asterisk indicates the significance of the difference between the indicated groups according to a Mann–Whitney test; * P <0.05. ( b ) Relative parasite 18S rRNA expression in the brain of AL and DR mice ( n =4 per diet group) 6 days after infection as determined by qPCR with a P value between AL and DR groups as indicated according to a Mann–Whitney test. ( c ) Naive, AL or DR mice ( n =4 per group) were injected with Evan’s blue and the leakage of the dye into the cerebral tissue representing disruption of BBB was qualitatively (left) and quantitatively (right) assessed on day 6 after infection. A representative experiment is shown. Asterisk indicates the significance of the difference between the indicated groups according to a Mann–Whitney test; * P <0.05. ( d ) Relative gene expression of chemokines, chemokine receptors and inflammatory markers as indicated in the brain on day 6 after infection of the indicated dietary group as measured by qPCR. Representative experiments with four mice per group are shown. Asterisks indicate the significance of the difference between AL and DR for a given gene according to a Mann–Whitney test; * P <0.05. ( e – g ) Numbers of total ( e ) and activated ( f , g ) CD4+ and CD8+ T lymphocytes with representative dot plots from brains of mice ( n =4 per group) of the indicated dietary groups on day 6 after infection following perfusion as determined by FACS. Asterisks indicate the significance of the difference between groups according to a Mann–Whitney test; * P <0.05. Values are means+s.e.m. Full size image To evaluate whether DR-mediated protection was associated with preservation of the BBB, we measured the accumulation of Evan’s blue in the brain of mice after 6 days of infection. Consistent with reduced ECM neuropathology, we observed significantly reduced leakage of the dye into brains of restricted mice as compared with the AL group ( Fig. 2c ). Relative mRNA expression of important chemokines in ECM, including CCL-5, CXCL-9 and CXCL-10, chemokine receptors CCR2 and CXCR3 (refs 17 , 25 , 26 , 27 , 28 , 29 , 30 ), and the cell surface adhesion marker ICAM-1 were also reduced in the brain upon DR on day 6 after infection ( Fig. 2d ). Inhibition of T-cell recruitment to the brain by DR Antigen-specific CD8+ T cells participate in ECM by promoting breakdown of BBB in the presence of parasitized RBCs [18] , [19] , [31] , [32] . To determine the effect of DR on T-cell recruitment to the brain, we quantified the number of CD4+ and CD8+ T cells in brains of perfused AL and DR mice by flow cytometry on day 6 after infection, coincident with the onset of neurological symptoms. Total numbers of CD4+ and CD8+ T cells, which are virtually undetectable in non-infected, or naive mice, were increased upon infection in AL mice by day 6; however, significantly less lymphocytes were detected in brains of DR mice compared with those of AL controls ( Fig. 2e ). Moreover, the number of CD4+ and CD8+ cells expressing activation markers CD69, lymphocyte function-associated antigen 1 (LFA-1) and/or granzyme B were significantly reduced in brains of restricted mice relative to AL controls ( Fig. 2f,g ). Taken together, these results strongly suggest that protection afforded by DR is multifactorial and mediated at least in part by reduced accumulation of infected RBCs in the brain, decreased recruitment of activated T cells and preservation of BBB integrity. Reduced sequestration and enhanced splenic clearance upon DR Accumulation, or sequestration, of parasitized RBCs in peripheral tissues is a strategy employed by Plasmodium parasites to avoid clearance in the spleen. Whole-body real-time in vivo imaging of luciferase-expressing P. berghei ANKA parasites [24] suggested an overall reduction in parasite burden, not only in brain, but also in major sequestering organs including the lung and white adipose tissue (WAT) on day 6 in DR mice relative to AL controls ( Fig. 3a ). To confirm these observations, mice were killed and perfused at different time points after infection, and luciferase activity measured in organ extracts. Parasite sequestration in the lung and WAT by day 6 after infection was significantly reduced in DR animals compared with AL controls ( Fig. 3b,c ). Parasitemia in blood, the single major source of overall parasite burden based on total luciferase activity corrected for volume, was similar in AL and DR until day 6 according to luciferase and fluorescence-activated cell sorting (FACS)-based measurements ( Supplementary Fig. 3A,B ). 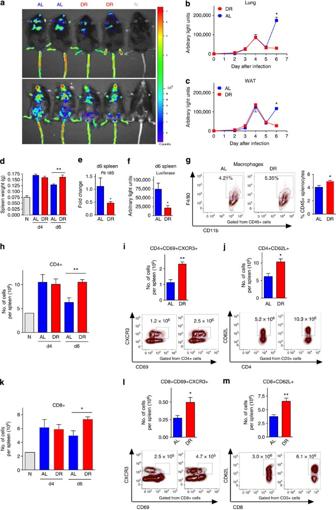Figure 3: Dietary restriction reduces total parasite sequestration and increases parasite spleen clearance. (a)In vivoimaging of parasite luciferase expression in live mice (dorsal view, top; ventral view, bottom) of the indicated diet group on day 6 after infection. A naive mouse (N) is shown as a control. (b,c) Parasite luciferase activity measured in extracts of lung (b) and WAT (c) over a time course after infection from a representative experiment withn=4 mice per dietary group per time point. Asterisks indicate the significance of the difference on day 6 after infection according to a Mann–Whitney test; *P<0.05. (d) Spleen weights of AL and DR mice (n=11–12 per group) on day 4 and day 6 after infection. Weights of spleens harvested from naive animals (N;n=6 per group) are shown as controls. Data are cumulative results of three independent experiments. Asterisks indicate the significance of the difference on the indicated day according to a Mann–Whitney test; **P=0.01. (e,f) Relative parasite 18S rRNA expression as determined by qPCR (e), and parasite luciferase activity (f) in spleens of AL and DR mice (n=5 per diet group) on day 6 after infection. Asterisks indicate the significance of the difference between groups according to a Mann–Whitney test; *P<0.05. (g) Percentages of splenic macrophages and representative dot plots from AL and DR mice on day 6 post infection. (h,k) Total numbers of splenic CD4+ (h), and CD8+ (k) T cells as measured by flow cytometry on days 4 and 6 (d4, d6) after infection in spleens of naive (N), AL and DR mice as indicated. (i,j,l,m) Total numbers of CD4+CD69+CXCR3+ (i), CD4+CD62L (j), CD8+CD69+CXCR3+ (l) and CD8+CD62L+ (m) T cells with representative dot plots from AL and DR mice measured on day 6 post infection. A representative experiment with five mice per dietary group is shown. Asterisks indicate the significance of the difference on the indicated day according to a Mann–Whitney test; *P<0.05. Values are means±s.e.m. Figure 3: Dietary restriction reduces total parasite sequestration and increases parasite spleen clearance. ( a ) In vivo imaging of parasite luciferase expression in live mice (dorsal view, top; ventral view, bottom) of the indicated diet group on day 6 after infection. A naive mouse (N) is shown as a control. ( b , c ) Parasite luciferase activity measured in extracts of lung ( b ) and WAT ( c ) over a time course after infection from a representative experiment with n =4 mice per dietary group per time point. Asterisks indicate the significance of the difference on day 6 after infection according to a Mann–Whitney test; * P <0.05. ( d ) Spleen weights of AL and DR mice ( n =11–12 per group) on day 4 and day 6 after infection. Weights of spleens harvested from naive animals (N; n =6 per group) are shown as controls. Data are cumulative results of three independent experiments. Asterisks indicate the significance of the difference on the indicated day according to a Mann–Whitney test; ** P =0.01. ( e , f ) Relative parasite 18S rRNA expression as determined by qPCR ( e ), and parasite luciferase activity ( f ) in spleens of AL and DR mice ( n =5 per diet group) on day 6 after infection. Asterisks indicate the significance of the difference between groups according to a Mann–Whitney test; * P <0.05. ( g ) Percentages of splenic macrophages and representative dot plots from AL and DR mice on day 6 post infection. ( h , k ) Total numbers of splenic CD4+ ( h ), and CD8+ ( k ) T cells as measured by flow cytometry on days 4 and 6 (d4, d6) after infection in spleens of naive (N), AL and DR mice as indicated. ( i , j , l , m ) Total numbers of CD4+CD69+CXCR3+ ( i ), CD4+CD62L ( j ), CD8+CD69+CXCR3+ ( l ) and CD8+CD62L+ ( m ) T cells with representative dot plots from AL and DR mice measured on day 6 post infection. A representative experiment with five mice per dietary group is shown. Asterisks indicate the significance of the difference on the indicated day according to a Mann–Whitney test; * P <0.05. Values are means±s.e.m. Full size image Reduced sequestration in the lung and WAT suggested enhanced clearance by the spleen in the DR group after day 4. Consistent with this, by day 6, spleen weights of DR animals were significantly greater than those of AL mice ( Fig. 3d ). Interestingly, despite greater spleen weights, luciferase activity as well as parasite 18S rRNA indicative of parasite burden were reduced in the spleens of DR relative to AL mice, possibly because of rapid disruption of parasites in phagolysosomal compartments of splenic macrophages and dendritic cells ( Fig. 3e,f ). Consistent with this possibility, the percentage of F4/80+CD11b+ macrophages in the total population of CD45+ splenocytes was significantly increased in the DR group on day 6 ( Fig. 3g ). Analysis of T lymphocytes was also consistent with an improved adaptive immune response to infection in DR animals ( Fig. 3h–m ). Although total numbers of CD4+ and CD8+ T cells from spleens of AL and DR mice were similar on day 4, both were significantly increased in DR animals on day 6 after infection ( Fig. 3h,k ) consistent with larger spleen size. Further analysis of CD4+ and CD8+ T-cell subpopulations revealed an increase in both activated T cells expressing CD69 and CXCR3 ( Fig. 3i,l ) and naive T cells expressing CD62L in the spleens of DR versus AL animals on day 6 of infection ( Fig. 3j,m ). Together these data suggest a scenario in DR mice on day 6 in which activated T cells remain in the spleen instead of migrating to the brain, while at the same time naive T cells and macrophages accumulate, allowing for increased clearance of infected RBCs. Leptin mediates pathology in ECM Leptin is a cytokine secreted mainly by adipocytes that increases in proportion to adiposity, and also upon exposure to pro-inflammatory stimuli including malaria infection [33] . While leptin signalling in the hypothalamus suppresses appetite, leptin signalling in immune cells promotes activation and secretion of pro-inflammatory cytokines [5] , [34] . Differences upon infection between AL and DR groups in appetite ( Fig. 1a,f ) and sequestration of parasitized RBCs in WAT ( Fig. 3a,c ) prompted us to consider leptin as a functional link between DR and ECM pathogenesis. Circulating leptin increased starting as early as day 2 after infection, peaking around days 6–7 in AL mice as previously reported [33] , but remained near baseline levels in DR mice ( Fig. 4a ). To test the requirement for leptin in ECM pathology, we used leptin-deficient ( ob/ob ) and leptin receptor-deficient ( db/db ) mice. Unlike WT mice, AL-fed ob/ob and db/db mice were protected against ECM while displaying similar parasitemias compared with WT mice ( Fig. 4b ). Protection in these hyperphagic models was unlikely due to increased adiposity, as obese WT mice with similar amounts of WAT were not protected ( Fig. 4b ; Supplementary Fig. 4A,B ). 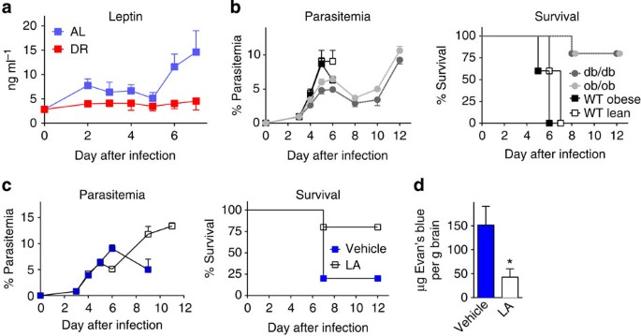Figure 4: Leptin is required for pathogenesis of ECM. (a) Serum leptin levels in AL-fed (AL) or restricted (DR) mice (n=4/ per group) over a time course after infection. (b) Wild-type mice (lean or obese as indicated) or mice deficient in leptin (ob/ob) or leptin receptor (db/db), all fed AL on a complete diet and infected on day 0 (n=5 per group).Peripheral parasitemia.The percentage of infected RBCs in circulation was assessed by flow cytometry on the indicated day after infection.Survival.Kaplan–Meier curves indicate a significant survival advantage in mice lacking leptin or leptin receptor (log-rank scoreP=0.0031) independent of adiposity. (c) Leptin antagonist (LA) prevented ECM in AL-fed WT mice. Peripheral parasitemia and survival curves for animals treated with vehicle or I mg kg−1per day of LA are shown (n=10 per group; log-rank scoreP=0.0089). (d) Vehicle or LA treated mice (n=5 per group) were injected with Evan's blue and the leakage of the dye into the cerebral tissue representing disruption of BBB was quantitatively assessed on day 6 after infection. Asterisk indicates the significance of the difference between the indicated groups according to a Mann-Whitney test; *P<0.05. Values are means±s.e.m. Figure 4: Leptin is required for pathogenesis of ECM. ( a ) Serum leptin levels in AL-fed (AL) or restricted (DR) mice ( n =4/ per group) over a time course after infection. ( b ) Wild-type mice (lean or obese as indicated) or mice deficient in leptin ( ob/ob ) or leptin receptor ( db/db ), all fed AL on a complete diet and infected on day 0 ( n =5 per group). Peripheral parasitemia. The percentage of infected RBCs in circulation was assessed by flow cytometry on the indicated day after infection. Survival. Kaplan–Meier curves indicate a significant survival advantage in mice lacking leptin or leptin receptor (log-rank score P =0.0031) independent of adiposity. ( c ) Leptin antagonist (LA) prevented ECM in AL-fed WT mice. Peripheral parasitemia and survival curves for animals treated with vehicle or I mg kg −1 per day of LA are shown ( n =10 per group; log-rank score P =0.0089). ( d ) Vehicle or LA treated mice ( n =5 per group) were injected with Evan's blue and the leakage of the dye into the cerebral tissue representing disruption of BBB was quantitatively assessed on day 6 after infection. Asterisk indicates the significance of the difference between the indicated groups according to a Mann-Whitney test; * P <0.05. Values are means±s.e.m. Full size image To further confirm the role of leptin in ECM pathology, we used a mutant leptin peptide that antagonizes leptin signalling in vivo [35] . AL mice treated with leptin antagonist peptide from day 1 to 6 after infection were significantly protected against neurological symptoms and death relative to vehicle-treated controls despite parasitemias similar to or higher than controls ( Fig. 4c ; Supplementary Movie 1 ). Moreover, leptin antagonist-treated mice were protected against BBB disruption as shown by a significant decrease in vascular permeability by day 6 post infection relative to AL-vehicle controls ( Fig. 4d ). Protection in antagonist-treated mice also correlated with maintenance of body weight and mitigated anorexic behaviour during infection ( Supplementary Fig. 4C ). Thus, our results clearly demonstrate a major role of leptin in ECM pathogenesis. DR protects against ECM via reduction of leptin Having established a requirement for leptin in ECM pathology, we next asked whether reduction of serum leptin contributed to protection afforded by DR. To test this, infected mice on DR were injected with up to 10 μg of recombinant mouse leptin twice a day from days 1 to 6 after infection. While vehicle-treated DR mice were protected, leptin abrogated this protection in a dose-dependent manner ( Fig. 5a ; Supplementary Fig. 5A ). Consistent with an important early role for DR in protection, leptin treatment only during the first 3 days after infection was sufficient to abrogate DR-mediated protection with respect to BBB damage, neurological symptoms and mortality ( Fig. 5a,b ; Supplementary Fig. 5A,B ). 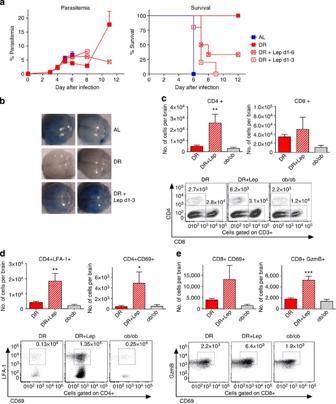Figure 5: Leptin abrogates benefits of dietary restriction. (a) Peripheral parasitemia and survival of mice in the indicated dietary groups (n=5 per group) infected on day 0 and treated with vehicle or recombinant leptin 10 μg twice daily on the indicated days. Log-rank scores indicated significant differences between DR and both DR/Leptin regimens (log-rank scoreP=0.029 d1–6;P=0.002 d1–3). (b) AL, DR or DR+leptin (d1–3) mice (n=4 per group) were injected with Evan’s blue and the leakage of the dye into the cerebral tissue representing disruption of BBB was quantitatively assessed on day 6 after infection. A representative experiment is shown. (c–e) Numbers of total (c) and activated (d,e) CD4+ and CD8+ T lymphocytes with representative dot plots, of DR, DR+leptin andob/obmice (n=5 per group) 6 days after infection following perfusion as determined by FACS. Asterisks indicate the significance of the difference according to a one-way analysis of variance (ANOVA) followed by Dunnett’s multiple comparison testing versus the DR group; *P<0.05. Values are means±s.e.m. Figure 5: Leptin abrogates benefits of dietary restriction. ( a ) Peripheral parasitemia and survival of mice in the indicated dietary groups ( n =5 per group) infected on day 0 and treated with vehicle or recombinant leptin 10 μg twice daily on the indicated days. Log-rank scores indicated significant differences between DR and both DR/Leptin regimens (log-rank score P =0.029 d1–6; P =0.002 d1–3). ( b ) AL, DR or DR+leptin (d1–3) mice ( n =4 per group) were injected with Evan’s blue and the leakage of the dye into the cerebral tissue representing disruption of BBB was quantitatively assessed on day 6 after infection. A representative experiment is shown. ( c – e ) Numbers of total ( c ) and activated ( d , e ) CD4+ and CD8+ T lymphocytes with representative dot plots, of DR, DR+leptin and ob/ob mice ( n =5 per group) 6 days after infection following perfusion as determined by FACS. Asterisks indicate the significance of the difference according to a one-way analysis of variance (ANOVA) followed by Dunnett’s multiple comparison testing versus the DR group; * P <0.05. Values are means±s.e.m. Full size image To assess the mechanism by which leptin abrogated DR-mediated protection, we analysed the migration and activation status of T cells in the brain of infected mice on DR with or without recombinant leptin treatment during the first 3 days of infection. AL-fed leptin-deficient ( ob/ob ) mice were included as an additional control. The abrogation of DR-mediated protection by recombinant leptin correlated with a significant increase in total ( Fig. 5c ) and activated ( Fig. 5d,e ) CD4+ and CD8+ T cells present in brains of treated mice on day 6 relative to DR or ob/ob mice. Thus, leptin add back in infected DR mice was sufficient to revert the protection afforded by food restriction and recapitulated immunological characteristics of ECM observed in AL-fed animals, strongly suggesting that DR-induced protection is mediated by decreased leptin production. Direct modulation of T-cell mTORC1 by leptin upon infection While DR mediates its beneficial effects at least in part by reducing activity of the nutrient/energy kinase mTORC1 (refs 11 , 14 , 36 , 37 , 38 ), immunomodulation by leptin in multiple cell types, including T lymphocytes and macrophages, occurs via activation of mTORC1 signalling [7] , [39] . To test mTORC1 activity in immune cells as the potential link between DR and leptin action in malarial infection, we looked at markers of mTORC1 activity in whole spleens, non-adherent splenocytes enriched for lymphocytes and adherent splenocytes enriched for macrophages and dendritic cells, isolated from AL or DR animals on day 3 after infection. Phosphorylation of the direct mTORC1 target S6K and/or its downstream target S6 were increased in AL mice relative to the DR group in spleens and enriched lymphocyte populations ( Fig. 6a,b ; Supplementary Fig. 6A ), while phosphorylation of the mTORC2 target NRDG1 was not consistently affected ( Supplementary Fig. 6B ). 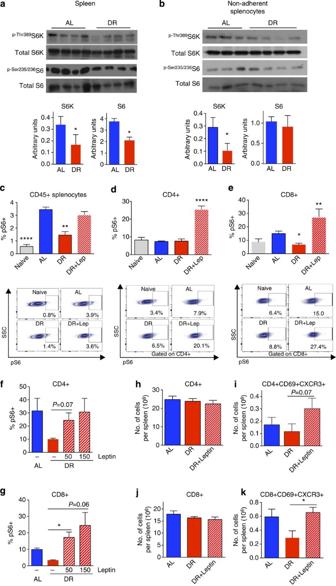Figure 6: Direct modulation of mTORC1 activity by leptin in T cells upon malarial infection. (a,b) Immunoblots of markers of mTORC1 signalling in spleens (a) or non-adherent splenocytes (b) of AL and DR animals on day 3 after infection. Quantitation of ratios of phosphorylated to total protein are presented below. Asterisks indicate the significance of the difference between AL and DR for the indicated protein according to a Mann–Whitney test; *P<0.05.n=4 mice per group. SeeSupplementary Fig. 6D,Efor full blots of the spleen and non-adherent splenocytes, respectively. (c–e) Analysis of S6 phosphorylation in splenocytes from naive or infected AL, DR or DR animals treated with leptin 1 h prior the experiment (DR+Lep) on day 3 post infection;n=4–5 animals per group. (c) Percentages of CD45+ splenocytes, CD4+ (d) and CD8+ (e) T cells positive for S6 phosphorylation are shown with corresponding representative dot plots. Asterisks indicate the significance of the difference between groups according to a one-way ANOVA followed by Dunnett’s multiple comparison testing versus the AL group; *P<0.05, **P<0.01, ****P<0.0001. (f,g)In vitroassessment of mTORC1 activity. Splenocytes from AL or DR mice on day 3 of infection were isolated and incubated for 1 h with or without leptin (50, 150 ng ml−1as indicated) and the percentage of CD4+ (f) and CD8+ (g) T cells with phosphorylated S6 assessed by FACS. (h–k) Functional consequences of leptin signalling and mTORC1 activation early in infection. Numbers of total CD4+ (h) and CD8+ (j) and activated CD4+CD69+CXCR3+ (i) and CD8+CD69+CXCR3+ (k) from spleens of AL, DR and DR+leptin (d1–3) mice (n=5 per group) on day 4 after infection as assessed by FACS. Asterisks indicate the significance of the difference between the indicated groups according to a Mann–Whitney test; *P<0.05. Values are means±s.e.m. Figure 6: Direct modulation of mTORC1 activity by leptin in T cells upon malarial infection. ( a , b ) Immunoblots of markers of mTORC1 signalling in spleens ( a ) or non-adherent splenocytes ( b ) of AL and DR animals on day 3 after infection. Quantitation of ratios of phosphorylated to total protein are presented below. Asterisks indicate the significance of the difference between AL and DR for the indicated protein according to a Mann–Whitney test; * P <0.05. n =4 mice per group. See Supplementary Fig. 6D,E for full blots of the spleen and non-adherent splenocytes, respectively. ( c – e ) Analysis of S6 phosphorylation in splenocytes from naive or infected AL, DR or DR animals treated with leptin 1 h prior the experiment (DR+Lep) on day 3 post infection; n =4–5 animals per group. ( c ) Percentages of CD45+ splenocytes, CD4+ ( d ) and CD8+ ( e ) T cells positive for S6 phosphorylation are shown with corresponding representative dot plots. Asterisks indicate the significance of the difference between groups according to a one-way ANOVA followed by Dunnett’s multiple comparison testing versus the AL group; * P <0.05, ** P <0.01, **** P <0.0001. ( f , g ) In vitro assessment of mTORC1 activity. Splenocytes from AL or DR mice on day 3 of infection were isolated and incubated for 1 h with or without leptin (50, 150 ng ml −1 as indicated) and the percentage of CD4+ ( f ) and CD8+ ( g ) T cells with phosphorylated S6 assessed by FACS. ( h – k ) Functional consequences of leptin signalling and mTORC1 activation early in infection. Numbers of total CD4+ ( h ) and CD8+ ( j ) and activated CD4+CD69+CXCR3+ ( i ) and CD8+CD69+CXCR3+ ( k ) from spleens of AL, DR and DR+leptin (d1–3) mice ( n =5 per group) on day 4 after infection as assessed by FACS. Asterisks indicate the significance of the difference between the indicated groups according to a Mann–Whitney test; * P <0.05. Values are means±s.e.m. Full size image We next sought to establish the cellular target of leptin action early in infection (day 3), and whether leptin can act directly on these cells. To this end, S6 phosphorylation status was measured by flow cytometry in specific splenocyte populations from naive or infected mice subject to AL feeding or DR with or without a single injection of recombinant leptin 1 h before harvest. mTORC1 activity increased upon infection in total splenocytes, macrophages and CD8+, but not CD4+, T cells from AL mice ( Fig. 6c–e ; Supplementary Fig. 6C ). DR reduced pS6 in total splenocytes, macrophages and CD8+ T cells, while leptin increased pS6 in total splenocytes, CD8+ and CD4+ T cells, but surprisingly not in macrophages ( Fig. 6c–e ; Supplementary Fig. 6C ), suggesting cell type specificity to the effects of leptin on mTORC1 signalling. To test for direct effects on T lymphocytes, single-cell suspensions of splenocytes were treated with leptin for one hour before pS6 flow cytometry. Leptin increased mTORC1 activity in CD4+ and CD8+ T cells in a dose-dependent manner ( Fig. 6f,g ). To further explore the functional consequences of leptin signalling and mTORC1 activation early in infection, splenic CD4+ and CD8+ T cells were further analysed for expression of activation markers including CXCR3 linked to mTORC1 activation in mice subject to DR with or without leptin treatment during the first 3 days of infection versus AL controls ( Fig. 6h–k ). Neither DR nor leptin injection had an effect on the number of splenic CD4+ nor CD8+ T cells by day 4 of infection ( Fig. 6h,j ). However, the effect of DR on CD8+ T cells double-positive for CD69 and CXCR3 was lost upon leptin treatment ( Fig. 6k ). A similar trend was observed in CD4+ T cells ( Fig. 6i ). Together, these results establish mTORC1 as a downstream target of leptin in T cells during ECM. mTORC1 inhibition protects via alteration of T-cell function To confirm the role of functional significance of mTORC1 activation in ECM pathology, we tested the ability of rapamycin to protect from ECM pathology. Rapamycin treatment of AL-fed mice over a range of doses during the first 3 days of infection had no effect on the ability of the parasite to grow ( Fig. 7a ), nor on mouse food intake or body weight ( Supplementary Fig. 7A,B ). However, even at the lowest dose, rapamycin treatment protected against the neurological complications of ECM ( Supplementary Movie 2 ) and significantly improved survival ( Fig. 7a ). Furthermore, treatment with rapamycin early in infection prevented accumulation of CD4+ and CD8+ T cells in the brain on day 6 after infection ( Fig. 7b ), including a specific reduction in the number of CD4+CD69+LFA-1+, CD8+CD69+LFA-1+ and CD8+CD69+granzyme B+ cells ( Fig. 7c–e ), consistent with a major role of mTORC1 in control of T-cell trafficking and effector function. While these data in no way rule out the potential importance of leptin action and mTORC1 signalling in other cell types, it demonstrates that pharmacological inhibition of leptin and mTORC1 signalling in the spleen early in infection can reduce trafficking of activated T cells to the brain later in infection, resulting in protection against ECM. 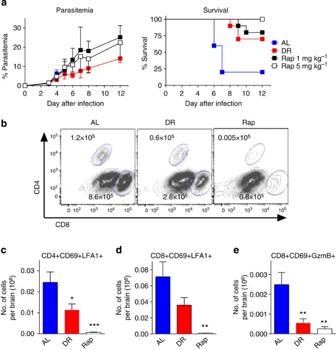Figure 7: Rapamycin treatment protects against ECM. (a) Parasitemia and survival of AL-fed mice treated with rapamycin on days 1–3 after infection with the indicated dose (n=10 per group). Vehicle-treated AL (n=5) and DR (n=10) mice served as controls. Log-rank scores indicated significant survival advantage upon rapamycin treatment relative to the vehicle-treated group (P=0.005 for low dose;P=0.0008 for high dose). (b) Representative dot plots of total CD4+ and CD8+ T cells from the brain of vehicle-treated AL, DR and rapamycin-treated AL (5 mg kg−1) mice on day 6 after infection. Corresponding cell numbers are indicated. (c–e) Activated triple-positive T-cell populations CD4+CD69+LFA-1+ (c), CD8+CD69+LFA-1+ (d) and CD8+CD69+granzyme B+ (e) from the brain on day 6 after infection of the indicated groups. Asterisks indicate the significance of the difference between according to a one-way ANOVA followed by Dunnett’s multiple comparison testing versus the AL group; *P<0.05, **P<0.01, ***P<0.001. Values are means±s.e.m. Figure 7: Rapamycin treatment protects against ECM. ( a ) Parasitemia and survival of AL-fed mice treated with rapamycin on days 1–3 after infection with the indicated dose ( n =10 per group). Vehicle-treated AL ( n =5) and DR ( n =10) mice served as controls. Log-rank scores indicated significant survival advantage upon rapamycin treatment relative to the vehicle-treated group ( P =0.005 for low dose; P =0.0008 for high dose). ( b ) Representative dot plots of total CD4+ and CD8+ T cells from the brain of vehicle-treated AL, DR and rapamycin-treated AL (5 mg kg −1 ) mice on day 6 after infection. Corresponding cell numbers are indicated. ( c – e ) Activated triple-positive T-cell populations CD4+CD69+LFA-1+ ( c ), CD8+CD69+LFA-1+ ( d ) and CD8+CD69+granzyme B+ ( e ) from the brain on day 6 after infection of the indicated groups. Asterisks indicate the significance of the difference between according to a one-way ANOVA followed by Dunnett’s multiple comparison testing versus the AL group; * P <0.05, ** P <0.01, *** P <0.001. Values are means±s.e.m. Full size image A model for the cellular and molecular mechanisms by which DR protects against ECM is presented in Fig. 8 . Differential food intake between DR and AL mice during the first 2–3 days of infection suppresses leptin production by adipocytes, resulting in a reduction in leptin-dependent mTORC1 activation in splenic T cells early in infection. In CD4+ and CD8+ T cells, inhibition of mTORC1 activity promotes homing of T cells to secondary lymphoid organs such as the spleen, decreasing the trafficking to inflamed tissues and decreasing the expression of activation markers and cytotoxic effector molecules. As a result, there is less homing of activated T cells to the brain, preventing the vicious cycle of T-cell-mediated endothelial damage facilitating further recruitment of activated T cells into the brain, and resulting in preservation of BBB integrity and protection from ECM neuropathology. Activated T cells instead remain in the spleen, while at the same time naive T cells and macrophages accumulate, allowing for increased clearance of infected RBCs. 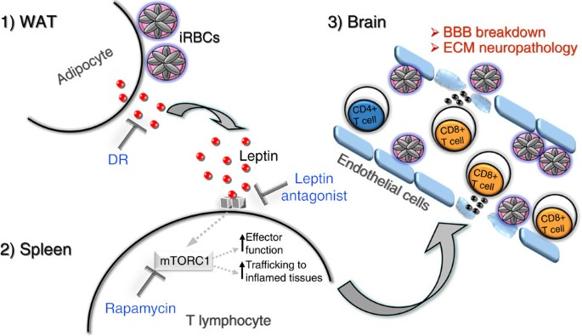Figure 8: Model for the role of leptin and mTORC1 in the pathogenesis of ECM. Sequestration of infected RBCs (iRBCs) to WAT activates leptin production by adipocytes early in infection. Increased circulating leptin activates mTORC1 in splenic T cells, leading to increased expression of chemokine receptors and effector molecules, and increasing the likelihood of trafficking to inflamed tissues such as the brain later in infection. DR mitigates leptin production by WAT early in infection. Suppression of the leptin–mTORC1 axis either by DR, leptin antagonist peptide or rapamycin results in significant inhibition of effector CD4+ and CD8+ T cells migration to the brain late in infection, preserving BBB function and reducing neuropathology, while enhancing T-cell function and parasite elimination in the spleen. Figure 8: Model for the role of leptin and mTORC1 in the pathogenesis of ECM. Sequestration of infected RBCs (iRBCs) to WAT activates leptin production by adipocytes early in infection. Increased circulating leptin activates mTORC1 in splenic T cells, leading to increased expression of chemokine receptors and effector molecules, and increasing the likelihood of trafficking to inflamed tissues such as the brain later in infection. DR mitigates leptin production by WAT early in infection. Suppression of the leptin–mTORC1 axis either by DR, leptin antagonist peptide or rapamycin results in significant inhibition of effector CD4+ and CD8+ T cells migration to the brain late in infection, preserving BBB function and reducing neuropathology, while enhancing T-cell function and parasite elimination in the spleen. Full size image In principle, modulation of diet can affect outcome of parasitic disease through effects on parasite growth and development, the host immune response or both. In ECM, protein restriction reduces parasite growth and development in vivo , thus preventing onset of neuropathology [40] , [41] . On the other hand, DR started 1 week before infection protects against ECM pathology without affecting parasite growth [42] . We confirmed this latter result and extended it in a number of important ways. First, we demonstrated that 40% DR starting as late as the day of infection resulted in protection, while DR beginning on day 2 after infection offered none. Interestingly, although there was an apparent reduction in protection when DR was started between 7 days before and co-incident with infection, this was probably the result of unusually high virulence in select experiments, rather than a biological effect. Consistent with the importance of DR within the first 2–3 days of infection, leptin treatment on the first 3 days of infection abrogated DR-mediated protection, while rapamycin treatment during the same period offered protection. Second, we showed that DR reduced parasite and leukocyte accumulation in the brain, protecting BBB integrity and preventing ECM neuropathology. Unresolved by our data, however, remains whether parasitized RBCs or cytotoxic CD8+ T cells are the initial trigger for BBB breakdown, as total parasite burden and recruitment of activated T lymphocytes to the brain were both reduced upon DR. Third, we showed that DR reduced parasite sequestration in highly sequestering tissues including lung and WAT after day 4 of infection, thus contributing to a reduction in overall parasite burden. Although the mechanism underlying reduced parasite sequestration was not directly addressed in our study, reduced sequestration upon DR could be secondary to reduced leukocyte recruitment to sequestering organs, as mice lacking T cells display defects in sequestration [19] . In the absence of data to suggest any effects of DR on parasite growth or development, we looked to enhanced splenic clearance of parasitized RBCs as the cause of the reduction in parasite burden. Unlike on day 4 after infection, when activated CD8+ T cells were reduced in spleens of DR animals, by day 6 numbers of both activated and naive CD4+ and CD8+ splenic T cells and macrophages were increased in DR animals, consistent with an increased capacity to clear parasitized RBCs relative to AL-fed mice. Furthermore, reduced Pb 18S and parasite-derived luciferase activity on day 6 after infection are consistent with enhanced splenic clearance of parasitized RBCs. We note, however, that because the persistence of Pb 18S and/or parasite-derived luciferase activity upon killing of parasites by macrophages is unknown, future experiments will be required to provide direct evidence of increased parasite clearance by the spleen upon DR, as well as to address the impact of DR on the ability to control parasite burden beyond day 12 of infection. Fourth, we demonstrated a novel requirement for leptin signalling in ECM pathology. Prior studies using leptin-deficient mice concluded that increased adiposity is protective against ECM [21] . This was puzzling, given that ECM is promoted by pro-inflammatory cytokines, and that hyperphagic leptin-deficient mice, much like obese wild-type mice, are in a chronic inflammatory state driven by nutrient excess. Our results indicate that the absence of leptin and leptin signalling, rather than adiposity per se , conferred protection, thus unlinking inflammation associated with obesity from leptin-dependent immune responses required for ECM neuropathology. Furthermore, we found that increasing leptin levels during the first 3 days of DR was sufficient to abrogate DR benefits and recapitulate the neuropathology of ECM observed in AL-fed animals, including an increase in activated CD4+ and CD8+ T cells in the brain on day 6 of infection. Because DR results in pleiotropic changes, these data do not imply that reduced leptin is the only mechanism of DR-mediated protection, nor do they in any way rule out direct or indirect effects of leptin on other cell types. For example, the potential effects of central leptin action on the hypothalamus in the progression of ECM, particularly in the later phase of infection when leptin levels are extremely high and AL animals display severe anorectic behaviour, is a fascinating question for future study. Nonetheless, our data identify leptin as a potential therapeutic host target against CM pathogenesis. Future studies will be required to test the role of WAT and parasite sequestration in early leptin production, as well as potential strategies targeting host adipokines in combating the deadly symptoms of CM. Finally, our data suggest mTORC1 in splenic CD4+ and CD8+ T cells as a relevant molecular target of increased leptin early in infection before the onset of neurological symptoms. mTORC1 has emerged as a crucial link between metabolism and immune function. It regulates CD8+ T-cell differentiation, activation, trafficking and function by controlling multiple transcription factors, including activation of T-bet, resulting in higher expression of CXCR3 and P-selectin ligands that are crucial for the trafficking of effector CD8+ T cells to inflamed tissues [9] , [10] , [43] . Importantly, CXCR3 has been shown to play an essential role in the induction of ECM pathology [27] , [28] , [30] . Of note, neutralization of leptin or leptin signalling and mTORC1 inhibition have similar effects on effector T cells [39] . Moreover, reminiscent of what we observed in DR-infected mice, mTORC1 inhibition can promote tolerance without compromising the ability of T cells to fight infections [44] . However, because inhibition of mTORC1 by rapamycin has pleiotropic effects on many cell types, including inhibition of leptin production by adipocytes [45] , as well as off-target effects on mTORC2 stability even upon short-term treatment [36] , future genetic experiments will be required to disentangle in which cell types mTORC1 activation is critical for ECM pathology. In conclusion, our study uncovers novel mechanisms by which brief changes in host diet can modulate the immunometabolism of the adaptive response to parasite infection via the host adipokine, leptin, with profound effects on disease outcome. Our data also identify two host factors, leptin and the nutrient/energy sensor mTORC1, as potential new targets against CM. Mice Wild-type and mutant ( ob/ob , db/db ) female C57BL/6J mice 8–10 weeks of age were purchased from Jackson Labs (Bar Harbor, ME, USA). Animals were housed four to five per cage and kept under standard laboratory conditions and allowed free access to water and food except as noted. All experiments were performed with the approval of the Harvard Medical Area animal care and use committee. Obese mice on a C57BL/6J background gained weight upon AL access to breeder’s chow in our animal facility. Food Mice were fed a purified diet (D124570B, Research Diets, New Brunswick, NJ, USA) with 72% calories from carbohydrate (sucrose, maltodextrin and corn starch), 18% calories from protein (casein) and 10% from fat (soybean oil and lard) supplemented with 15 mg of p -amino benzoic acid per 100 g of food. Powder diets were mixed with 1 l kg −1 diet of hot water containing 2% agar; the cooled mixture was given daily to mice either on an AL basis or restricted to a percentage of that eaten by the AL group (DR). Malaria infection Cryopreserved transgenic P. berghei ANKA parasites expressing luciferase/green fluorescent protein under a constitutive promoter [24] were thawed and passaged once in vivo before being used to infect experimental mice with 0.5 million parasitized RBCs/mouse by tail vein injection. Parasites from peripheral blood were stained with SYTO16 and the percentage of infected cells was calculated by flow cytometry [46] . The percentage of each parasite stage in peripheral blood was scored microscopically from fixed and Giemsa-stained blood smears. Individual mouse weights and food intake per cage were calculated daily. Parasite accumulation/sequestration Infected mice were killed on the indicated day and perfused with cold PBS intracardially. The organs were harvested, weighed and homogenized in an equal volume per mg tissue of luciferase activity assay buffer (Invitrogen). Blood luciferase activity was measured from 10 μl of whole blood in 100 μl of buffer. Equal volumes were mixed with luciferin substrate and measured in a 96-well luminometer (Biotek Synergy 2). For in vivo imaging, infected mice were anaesthetised and injected with luciferin, and luciferase activity detected with the IVIS Lumina In Vivo Imaging System. Serum and blood analyses Blood glucose was measured from fresh blood with an Easy Check Diabetes Meter Kit (Home Aid Diagnostics). Amino-acid concentrations were analysed using mass spectrometry. Leptin concentration in blood serum was measured with ELISA (mouse leptin, R&D systems) following the manufacturer’s instructions. Haematocrit, platelets and total leukocytes from fresh whole blood were measured on a Hemavet multispecies haematology system (Drew Scientific). Brain vascular permeability Day 6 infected mice were injected intravenously with 200 μl of PBS-2% Evans blue, killed 1 h later and perfused intracardially with cold PBS. Their brains were harvested, weighed and placed in 2 ml 100% formamide (Merck) for 48 h at 37 °C. Absorbance of the formamide supernatant was measured at 620 nm. Evans blue concentration was calculated from a standard curve and results expressed as microgram of Evans blue per gram of brain tissue. Isolation and analysis of leukocyte populations Brains and spleens were harvested at the indicated days after perfusion with cold PBS. Spleen single-cell suspensions were prepared by homogenization through a 70-μm cell strainer (BD Falcon). Brains were digested with 50 U ml −1 of type II and IV collagenase (Gibco, Invitrogen) in RPMI, and mononuclear cells isolated on a 33% Percoll density gradient (GE Healthcare). After lysing RBCs and determining the total cell concentration, cells were incubated with an FcR blocker (Mitenyi Biotech), labelled for extracellular antigens, fixed with 4% paraformaldehyde and stained for intracellular markers using the Cytofix/Cytoperm kit (BD Biosciences) following the manufacturer’s instructions. For assessment of mTORC1 signalling, cells were incubated in DPBS containing 0.5% BSA, 2 mM EDTA, 5 mM β-glycerophosphate and 20 mM NaF during extracellular antigen labelling, fixed with 4% paraformaldehyde, labelled with a 1:100 dilution of Alexa 488 rabbit anti-pS6 (Cell Signaling Technologies, Baverly, USA) and resuspended in 0.2% saponin in DPBS. Single fluorochrome-labelled cells were used to compensate for spectral overlap. Isotype-matched fluorescence minus one controls were used to set gate cutoffs. Acquisition was performed using a BD Fortessa and data analysed using FlowJo (Tree Star Inc.). Histology Mice were perfused intracardially with PBS on the indicated day. Brains fixed in 4% paraformaldehyde in PBS were embedded in paraffin, cut and stained with haematoxylin and eosine (H&E) before analysis. Quantitative real-time PCR Total RNA was extracted from frozen tissue with RNA Bee (Qiagen, Valencia, CA, USA), and with the Qiagen RNeasy mini Kit (Qiagen) for sorted cells. Hexamer-primed cDNA was synthesized with the Verso cDNA Kit (Thermo Scientific) according to the manufacturer’s instructions. Quantitative real-time PCR was performed with an MyIQ (Bio-Rad) using SYBR Green. Relative expression was calculated with the ΔΔ C t method. cDNA expression of each sample was standardized to HPRT. Each sample was tested in duplicate at least twice. Primer sequences used: CCL-5 , fwd: 5′-GCAAGTGCTCCAATCTTGCA-3′; rev: 5′-CTTCTCTGGGTTGGCACACA-3′. CXCL-9 , fwd: 5′-GCCATGAAGTCCGCTGTTCT-3′; rev: 5′-GGGTTCCTCGAACTCCACACT-3′. CXCL-10 , fwd: 5′-GACGGTCCGCTGCAACTG-3′; rev: 5′-GCTTCCCTATGGCCCTCATT-3′. CCR2 , fwd: 5′-GAAGGAGGGAGCAGTGTGTACAT-3′; rev: 5′-CCCCCACATAGGGATCATGA-3′. CCR5 , fwd: 5′-GGCCATGCAGGCAACAG-3′; rev: 5′-TCTCCAACAAAGGCATAGATGACA-3′. CXCR3 , fwd: 5′-AATGCCACCCATTGCCAGTAC-3′; rev: 5′-AGCAGTAGGCCATGACCAGAAG-3′. ICAM-1 , fwd: 5′-GCCTCCGGACTTTCGATCTT-3′; rev: 5′-GTCAGGGGTGTCGAGCTTTG-3′. IFN-γ , fwd: 5′-CAGCAACAGCAAGGCGAAA-3′; rev: 5-GCTGGATTCCGGCAACAG-3′. Pb18S , fwd: 5′-AAGCATTAAATAAAGCGAATACATCCTTAC-3′; rev: 5′-GGAGATTGGTTTTGACGTTTATGTG-3′. In vivo leptin, leptin antagonist and rapamycin treatments One, three or ten micrograms of recombinant mouse leptin (R&D Systems) was administered twice a day by intraperitoneal (i.p.) injection to infected mice on DR from day 1 to day 6 or from day 1 to day 3 of infection. In some experiments, DR mice on day 3 post infection were injected i.p. with recombinant leptin once, and splenocytes isolated 1 h later. A pegylated super mouse leptin antagonist PESLAN-1 (Protein Laboratories, Rehovot) was administered i.p. to AL-infected mice at 0.25, 0.75 or 1 mg kg −1 per day from day 1 to day 6 of infection. Rapamycin (LC Laboratories, Woburn, MA, USA) was administered i.p. to AL-infected mice at 1 or 5 mg kg −1 per day on days 1–3 of infection. In vitro leptin and rapamycin treatments Splenocytes isolated from AL and DR mice on day 3 post infection were incubated for 1 h with serum-free DMEM alone or containing recombinant leptin at concentrations of 50 or 150 ng ml −1 or rapamycin at 100 nM (for AL cells only). Cells were then stained with specific antibodies for assessment of mTORC1 signalling as described above. Body composition Fat mass was assessed by noninvasive nuclear magnetic resonance (NMR) in awake animals (EchoMRI, Echo Medical Systems) on the day of infection. Immunoblots NP-40 extracts of snap-frozen spleens or primary adherent or non-adherent splenocytes were separated by SDS–PAGE, transferred to nitrocellulose and stained with the following antibodies (Cell Signaling Technologies) at a 1:1,000 dilution: Rb anti-β-Actin, Rb anti-total p70 S6K, Rb anti-phospho p70 S6K (Thr389), mouse anti-total S6, Rb anti-phospho S6 (Ser235/336 and Ser240/244) for mTORC1 signalling, and with phospho NGRD1 from Cell Signaling as well for mTORC2 signalling. Statistics Data are expressed as mean±s.e.m. unless indicated otherwise. Statistical analyses were performed in GraphPad Prism with Mann–Whitney, one-way analysis of variance or Kaplan–Meier survival analysis tests as indicated. How to cite this article : Mejia, P. et al. Dietary restriction protects against experimental cerebral malaria via leptin modulation and T-cell mTORC1 suppression. Nat. Commun. 6:6050 doi: 10.1038/ncomms7050 (2015).